Vimentin regulates activation of the NLRP3 inflammasome Activation of the NLRP3 inflammasome and subsequent maturation of IL-1β have been implicated in acute lung injury (ALI), resulting in inflammation and fibrosis. We investigated the role of vimentin, a type III intermediate filament, in this process using three well-characterized murine models of ALI known to require NLRP3 inflammasome activation. We demonstrate that central pathophysiologic events in ALI (inflammation, IL-1β levels, endothelial and alveolar epithelial barrier permeability, remodelling and fibrosis) are attenuated in the lungs of Vim −/− mice challenged with LPS, bleomycin and asbestos. Bone marrow chimeric mice lacking vimentin have reduced IL-1β levels and attenuated lung injury and fibrosis following bleomycin exposure. Furthermore, decreased active caspase-1 and IL-1β levels are observed in vitro in Vim −/− and vimentin-knockdown macrophages. Importantly, we show direct protein–protein interaction between NLRP3 and vimentin. This study provides insights into lung inflammation and fibrosis and suggests that vimentin may be a key regulator of the NLRP3 inflammasome. The cytoskeleton comprises microfilaments, microtubules and intermediate filaments (IFs) [1] . Vimentin is the most abundant IF protein and has a critical role in stabilizing intracellular architecture [2] . Until recently, the importance of vimentin remained elusive because vimentin knockout ( Vim −/− ) mice displayed a relatively normal phenotype [3] . However, a thorough characterization of Vim −/− mice under stress conditions revealed prominent abnormalities [4] , [5] , [6] , complementing the metabolic, signalling and regulatory abnormalities displayed by patients with IF-related diseases and mice expressing functional mutations in IFs [2] , [7] , [8] , [9] , [10] . Recently, evidence to support a role for IFs as scaffolds for macromolecular complexes involved in critical cell signalling functions was reported [11] , [12] . In this study, we demonstrate that vimentin is required for the activation of the NLRP3 (NACHT, LRR and PYD domains-containing protein 3) inflammasome, a macromolecular complex that orchestrates early inflammatory responses of the innate immune system. The NLRP3 inflammasome is activated in response to a broad spectrum of infectious agents known to cause acute lung injury (ALI), including the bacterial pathogens Staphylococcus aureus, Pseudomonas aeruginosa and Mycobacterim tuberculosis [13] , [14] , [15] and viral pathogens such as influenza A virus [16] . The wide range of pathogens known to activate the NLRP3 inflammasome suggests that NLRP3 indirectly senses microbes by probing for host-derived danger-associated molecular patterns that are produced or released after cellular or tissue injury [17] , [18] . For example, uric acid released from cells exposed to bleomycin triggers the NLRP3 inflammasome, leading to maturation of interleukin 1β (IL-1β) and inflammation [19] . In both human patients and animals treated with bleomycin, IL-1β released from injured cells results in production of the pro-fibrotic cytokine transforming growth factor β (TGF-β), which contributes to the development of pulmonary fibrosis [20] . In addition, exposure to crystalline particles such as asbestos and silica also cause pulmonary fibrosis [21] that is regulated by the NLRP3 inflammasome [22] , [23] . The NLRP3 inflammasome must be tightly regulated to avoid deleterious effects from the wide array of pathogens, pathogen-associated molecular patterns, danger-associated molecular patterns and environmental irritants, which are known to trigger its activation. Unlike other inflammasome-associated Nod-like receptor (NLR) proteins, NLRP3 is expressed at very low levels in naive macrophages. Activation of the NLRP3 inflammasome requires two distinct pro-inflammatory stimuli. In the first step, Toll-like receptor (TLR) signalling activates NF-κB and upregulates NLRP3 and pro-IL-1β [24] . The second step involves the assembly of the multiprotein complex, which induces self-cleavage of caspase-1, which in turn mediates the cleavage of pro-IL-1β into its biologically active form [25] . The mechanism by which the inflammasome is ultimately activated is still a subject of intensive research. We postulate that vimentin is required for NLRP3 inflammasome assembly and activation. The experiments described below use three well-established rodent models of NLRP3 inflammasome activation and result in increased levels of biologically active IL-1β that contribute to lung injury. Our data suggest that the IF protein vimentin may act as an additional checkpoint to control the NLRP3 inflammasome. Vimentin deficiency suppresses inflammation and injury Lipopolysaccharide (LPS) is a potent inducer of inflammation and a known NLRP3 inflammasome activator [26] , [27] , [28] . To determine whether vimentin is important in the inflammatory response, wild-type (WT) and vimentin knockout ( Vim −/− ) mice were subjected to a lethal dose of LPS, which induces both pro-inflammatory cytokine expression and a systemic inflammatory response that is associated with significant mortality. Wild-type mice displayed about a threefold increase in mortality compared with Vim −/− mice. Vim −/− mice had a median survival of 138 h, whereas WT animals had a median survival of ~40 h ( Fig. 1a ). Surviving Vim −/− mice exhibited mild lethargy, coat ruffling, febrile shaking and eye watering but recovered by day 7. 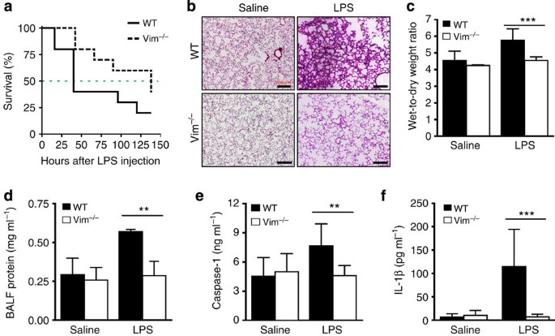Figure 1: Vimentin is required for ALI and inflammasome activation in response to LPS. (a) Survival of WT andVim−/−mice subjected to a lethal dose of LPS (80 mg kg−1, intraperitoneally) was measured and compared. The survival curves were analysed using the log rank test, which calculates the chi-square (χ2) for each event time for each group and sums the results. The summed results for each group were added to derive the ultimate chi-square to compare the full curves of each group. The log rank test for the entire data set wasP=0.001. (b–f) WT andVim−/−mice were challenged with a sublethal dose of LPS and markers of ALI were measured after 48 h, as assessed by H&E staining (scale bar, 200 μm) (b); by wet-to-dry lung weight ratio (c); and by protein content in the BALF (d). Inflammasome activation was measured by ELISA for caspase-1 (e) or IL-1β (f) in BALF fromVim−/−and WT mice. Data inb–eare from three independent experiments ofn=6–8 animals per group and presented as mean±s.d. **P<0.001, ***P<0.0001 relative to WT versusVim−/−, by one-way analysis of variance with a correction provided by the Bonferroni multiple comparisons test. Figure 1: Vimentin is required for ALI and inflammasome activation in response to LPS. ( a ) Survival of WT and Vim −/− mice subjected to a lethal dose of LPS (80 mg kg −1 , intraperitoneally) was measured and compared. The survival curves were analysed using the log rank test, which calculates the chi-square ( χ 2 ) for each event time for each group and sums the results. The summed results for each group were added to derive the ultimate chi-square to compare the full curves of each group. The log rank test for the entire data set was P =0.001. ( b – f ) WT and Vim −/− mice were challenged with a sublethal dose of LPS and markers of ALI were measured after 48 h, as assessed by H&E staining (scale bar, 200 μm) ( b ); by wet-to-dry lung weight ratio ( c ); and by protein content in the BALF ( d ). Inflammasome activation was measured by ELISA for caspase-1 ( e ) or IL-1β ( f ) in BALF from Vim −/− and WT mice. Data in b – e are from three independent experiments of n =6–8 animals per group and presented as mean±s.d. ** P <0.001, *** P <0.0001 relative to WT versus Vim −/− , by one-way analysis of variance with a correction provided by the Bonferroni multiple comparisons test. Full size image To study whether vimentin affects LPS-induced inflammation and ALI, we used a sublethal dose of LPS, as previously described [29] , [30] . Histopathological examination showed that lungs of LPS-treated WT mice had more severe alveolar damage characterized by interstitial oedema and more fluid and debris in the airspace than in LPS-treated Vim −/− mice ( Fig. 1b ). Wild-type mice exposed to LPS exhibited an increase in wet-to-dry lung weight ratio and total protein concentration in the bronchoalveolar lavage fluid (BALF), whereas Vim −/− mice failed to exhibit such an increase ( Fig. 1c,d ). Exposure to LPS is followed by large increases in immune cells in the airspace [29] , [30] . Therefore, to further characterize the nature of immune cell recruitment into the lungs, we performed a systematic flow cytometric analysis of whole-lung lysates [31] . No differences were observed in the myeloid cell population between WT and Vim −/− mice treated with saline ( Supplementary Fig. 1a ). As expected, both WT and Vim −/− mice challenged with LPS had significant increases in neutrophils and moderate increases in macrophages compared with saline-treated animals ( Supplementary Fig. 1a ); no differences were observed between WT and Vim −/− mice challenged with LPS ( Supplementary Fig. 1a ). These data suggest that the protection from the LPS-induced increase in alveolar capillary barrier permeability observed in Vim −/− mice was not associated with impaired recruitment of inflammatory cells to the lung. LPS induces rapid production and release of pro-inflammatory cytokines and chemokines, which are sufficient to induce lung inflammation and ALI in mice and humans [32] . When we exposed WT and Vim −/− mice to LPS for 24 h, significantly more caspase-1 and mature IL-1β were found in BALF from WT mice than in Vim −/− mice ( Fig. 1e,f ). Furthermore, whole-lung homogenates prepared from WT and Vim −/− mice exposed to LPS had increased levels of IL-1β messenger RNA (mRNA, Supplementary Fig. 1b ). These data suggest that vimentin is not involved in the TLR-mediated NF-κB activation and upregulation of pro-IL-1β and NLRP3 (refs 26 , 27 , 28 ). Rather, vimentin must be required for the second step in LPS-induced caspase-1 activation and IL-1β maturation via the NLRP3 inflammasome. Vimentin required for asbestos-induced injury and fibrosis The NLRP3 inflammasome has been implicated in the pathological increase of IL-1β production in a variety of pulmonary inflammatory diseases that lead to fibrosis, including asbestosis [21] , [22] , [23] . In a model of asbestosis, we sought to determine whether Vim −/− mice showed diminished cytokine production and whether these animals were protected from lung injury and pulmonary fibrosis. Wild-type and Vim −/− mice were exposed to crocidolite asbestos or an inert particle, titanium dioxide (TiO 2 ); markers of injury, inflammation, cytokine production and fibrosis were assessed. Confirming previous reports [22] , [23] , asbestos-exposed mice had increased total cell numbers in BALF compared with TiO 2 -exposed animals. However, significantly fewer cells were recruited to the lungs of Vim −/− mice after asbestos exposure ( Fig. 2a ). Additional analysis of immune cell recruitment into the lungs of WT and Vim −/− mice was performed by fluorescence-activated cell sorting analysis of whole-lung lysates ( Supplementary Fig. 2a ). Wild-type mice had profound inflammatory cell infiltrates following exposure to asbestos as observed by haematoxylin and eosin (H&E) staining; in contrast Vim −/− mice showed reduced inflammation ( Supplementary Fig. 2b ). Wild-type mice exhibited an increase in total protein concentration in BALF, whereas Vim −/− mice failed to exhibit such an increase ( Fig. 2b ). The reduction in inflammation in Vim −/− mice exposed to asbestos was associated with reduced levels of caspase-1 and IL-1β in BALF compared with WT mice ( Fig. 2c,d ). These data suggest that vimentin is required for asbestos-mediated activation of the NLRP3 inflammasome (step 2), but not for NF-κB activation and upregulation of pro-IL-1β and NLRP3 (step 1). Furthermore, we observed that WT mice exposed to asbestos develop pulmonary fibrosis, as assessed by Masson trichrome and Picrosirius red stain (a dye that binds specifically to collagen fibrils, Fig. 2e ) and Sircol assay ( Fig. 2f ). Vimentin deficiency prevented pulmonary fibrosis, as no significant increase in collagen deposition was observed in Vim −/− mice ( Fig. 2e,f ). Collectively, these results demonstrate that loss of vimentin prevents asbestos-induced collagen deposition and fibrosis. 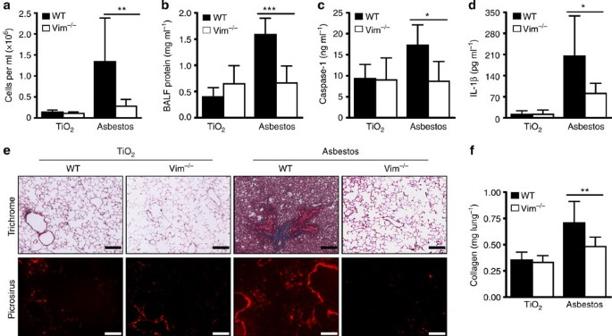Figure 2: Vimentin deficiency prevents asbestos-induced lung injury and fibrosis. WT andVim−/−mice were treated with PBS containing either 200 μg of asbestos crocidolite or the control particle titanium dioxide (TiO2), intratracheally. Markers of inflammation and fibrosis were assessed 3 and 6 weeks after instillation, respectively. (a) Total cell count (macrophages, neutrophils, eosinophils, erythrocytes and lymphocytes ) and (b) protein levels were assessed in BALF collected fromVim−/−mice 3 weeks after asbestos administration. Inflammasome activation in WT andVim−/−mice was measured by ELISA for caspase-1 (c) and IL-1β (d) levels in BALF at the same time point. Collagen deposition was evaluated in asbestos-treatedVim−/−and WT mice by Masson’s trichrome and Picrosirius red staining of lung slices (e; scale bar, 200 μm) and by measuring total collagen content by Sircol assay (f). Data are from two independent experimentsn=6–8 animals per group, and presented as mean±s.d. *P<0.05, **P<0.001, relative to WT versusVim−/−, by one-way analysis of variance with a correction provided by the Bonferroni multiple comparisons test. Figure 2: Vimentin deficiency prevents asbestos-induced lung injury and fibrosis. WT and Vim −/− mice were treated with PBS containing either 200 μg of asbestos crocidolite or the control particle titanium dioxide (TiO 2 ), intratracheally. Markers of inflammation and fibrosis were assessed 3 and 6 weeks after instillation, respectively. ( a ) Total cell count (macrophages, neutrophils, eosinophils, erythrocytes and lymphocytes ) and ( b ) protein levels were assessed in BALF collected from Vim −/− mice 3 weeks after asbestos administration. Inflammasome activation in WT and Vim −/− mice was measured by ELISA for caspase-1 ( c ) and IL-1β ( d ) levels in BALF at the same time point. Collagen deposition was evaluated in asbestos-treated Vim −/− and WT mice by Masson’s trichrome and Picrosirius red staining of lung slices ( e ; scale bar, 200 μm) and by measuring total collagen content by Sircol assay ( f ). Data are from two independent experiments n =6–8 animals per group, and presented as mean±s.d. * P <0.05, ** P <0.001, relative to WT versus Vim −/− , by one-way analysis of variance with a correction provided by the Bonferroni multiple comparisons test. Full size image Vimentin required for bleomycin-induced injury and fibrosis Bleomycin is one of the best characterized rodent models of pulmonary fibrosis [33] ; intratracheal delivery of the drug causes severe ALI, which is followed by clearance of alveolar inflammatory cells, fibroblast proliferation and increased collagen deposition [34] . Moreover, bleomycin-induced fibrosis has been shown to be dependent on the NLRP3 inflammasome [35] . WT and Vim −/− mice were exposed to bleomycin for 5 days. WT mice displayed intense lung inflammation as assessed by H&E staining ( Fig. 3a ), increased wet-to-dry lung weight ratio ( Fig. 3b ), and increased protein concentration in BALF ( Fig. 3c ). All of these end points were significantly attenuated in Vim −/− mice ( Fig. 3a–c ). Exposure to bleomycin resulted in a large increase in immune cells in the airspace of both WT and Vim −/− mice as assessed by flow cytometric analysis of whole-lung lysates ( Supplementary Fig. 3a ). Vim −/− mice failed to exhibit an increase in caspase-1 ( Fig. 3d ) and IL-1β ( Fig. 3e ) in BALF following the exposure to bleomycin; in contrast, WT mice showed a robust activation of caspase-1 and production of mature IL-1β ( Fig. 3d,e ). As a pro-inflammatory cytokine, macrophage-produced IL-1β is known to induce production of interleukin 6 (IL-6). We observed that WT mice, but not Vim −/− mice, had increased levels of IL-6 following the exposure to bleomycin ( Fig. 3f ). TGF-β1 is a critical mediator of remodelling and fibrotic responses in the lung. Total TGF-β1 was detected after activation in BALF from WT mice 5 days following the exposure to bleomycin, but remained at the baseline level in BALF from Vim −/− mice ( Fig. 3g ). No significant difference was observed between WT and Vim −/− mice in NLRP3 inflammasome-independent cytokines TNF-α and MCP-1 ( Fig. 3h,i ). Interestingly, IL-1β mRNA levels were increased in the lungs of both WT and Vim −/− mice following the exposure to bleomycin ( Supplementary Fig. 3b ). 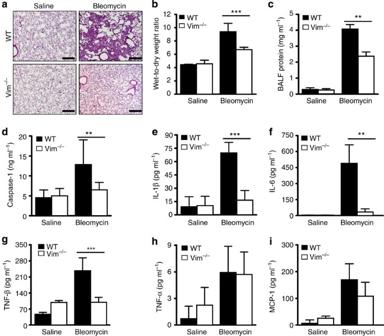Figure 3: Vimentin is required for bleomycin-induced lung injury. WT andVim−/−mice were treated with either bleomycin (0.07 U ml−1, intratracheally) or saline and assessed on day 5. (a) Bleomycin-induced lung injury was assessed by histological examination of H&E staining of lung tissue (original magnification × 10; scale bar, 200 μm), (b) lung wet-to-dry weight ratio and (c) protein levels in BALF. Inflammasome activation was assessed by ELISA for levels of caspase-1 (d) and IL-1β (e) in BALF.Levels of IL-6 (f) and TGF-β1 (g) in BALF were assessed by ELISA. Inflammasome-independent cytokines MCP-1 (h) and TNF-α (i) were measured in WT andVim−/−mice. Images inaare representative of four to six animals per condition. Data inb–iare means±s.d. from two independent experimentsn=4–6 animals per group. **P<0.001, ***P<0.0001, relative to WT versusVim−/−, by one-way analysis of variance with a correction provided by the Bonferroni multiple comparisons test. Figure 3: Vimentin is required for bleomycin-induced lung injury. WT and Vim −/− mice were treated with either bleomycin (0.07 U ml −1 , intratracheally) or saline and assessed on day 5. ( a ) Bleomycin-induced lung injury was assessed by histological examination of H&E staining of lung tissue (original magnification × 10; scale bar, 200 μm), ( b ) lung wet-to-dry weight ratio and ( c ) protein levels in BALF. Inflammasome activation was assessed by ELISA for levels of caspase-1 ( d ) and IL-1β ( e ) in BALF.Levels of IL-6 ( f ) and TGF-β1 ( g ) in BALF were assessed by ELISA. Inflammasome-independent cytokines MCP-1 ( h ) and TNF-α ( i ) were measured in WT and Vim −/− mice. Images in a are representative of four to six animals per condition. Data in b – i are means±s.d. from two independent experiments n =4–6 animals per group. ** P <0.001, *** P <0.0001, relative to WT versus Vim −/− , by one-way analysis of variance with a correction provided by the Bonferroni multiple comparisons test. Full size image Bleomycin exposure results in chronic inflammation and progressive pulmonary fibrosis [19] , [35] . The role of vimentin in pulmonary fibrosis was examined 21 days following the administration of bleomycin. The lung architecture was similar for saline-treated WT and Vim −/− mice, but in WT mice bleomycin induced extensive fibrotic areas with abundant collagen production, as assessed by Masson trichrome stain ( Fig. 4a and Supplementary Fig. 4a ). Cellular infiltrates, alveolar wall destruction and collagen deposition were significantly reduced in Vim −/− mice. Similarly, we observed increases in collagen deposition in bleomycin-treated WT mice by staining with Picrosirius red ( Fig. 4b ). In contrast, there was virtually no collagen deposition in the lungs of Vim −/− mice ( Fig. 4b ). Lung collagen concentrations, as assessed by Sircol assay, were 0.57±0.09 and 0.31±0.03 mg per lung in bleomycin-treated WT and Vim −/− mice, respectively ( Fig. 4d ). 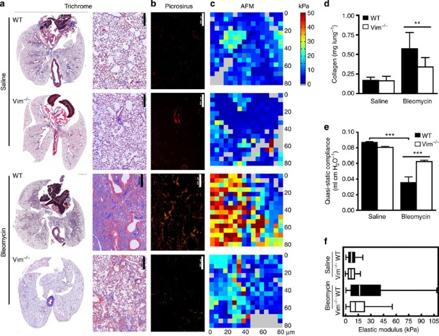Figure 4: Bleomycin-induced lung injury and fibrosis are prevented in the absence of vimentin. Shown is the histology of mice lungs 21 days following intratracheal instillation of bleomycin or PBS. Masson trichrome (a) and Picrosirius Red (b) stains for collagen. Original magnification for overview mosaics, × 5. Enlargements were taken with a × 40 objective (scale bar, 200 μm). (c) Representative elastographs from AFM micro-indentation of lung tissue from WT andVim−/−animals. The colour bar indicates elastic modulus,E. The darkest red corresponds to elastic modulus values of 50 kPa and above. The data represent 256 indentations per region, with at least two regions per tissue section from at least three mice per group. (d) Collagen content in lungs from WT andVim−/−mice assessed by Sircol assay. (e) Mice were ventilated 21 days after intratracheal instillation of bleomycin or PBS. Shown are quasi-static compliance measurements of WT andVim−/−lungs. (f) Elastic modulus frequency plot obtained from live, unfixed lung tissue of saline and bleomycin-treated WT andVim−/−animals. Microindentation data were fit using the Hertz model to acquire the elastic modulus of regions of lung tissue. Images ina–brepresent data obtained from at least three animals per group; data shown ind–eare mean±s.d. of at least five animals. **P<0.001, ***P<0.0001 relative to WT versusVim−/−, by one-way analysis of variance with a correction provided by the Bonferroni multiple comparisons test. Figure 4: Bleomycin-induced lung injury and fibrosis are prevented in the absence of vimentin. Shown is the histology of mice lungs 21 days following intratracheal instillation of bleomycin or PBS. Masson trichrome ( a ) and Picrosirius Red ( b ) stains for collagen. Original magnification for overview mosaics, × 5. Enlargements were taken with a × 40 objective (scale bar, 200 μm). ( c ) Representative elastographs from AFM micro-indentation of lung tissue from WT and Vim −/− animals. The colour bar indicates elastic modulus, E . The darkest red corresponds to elastic modulus values of 50 kPa and above. The data represent 256 indentations per region, with at least two regions per tissue section from at least three mice per group. ( d ) Collagen content in lungs from WT and Vim −/− mice assessed by Sircol assay. ( e ) Mice were ventilated 21 days after intratracheal instillation of bleomycin or PBS. Shown are quasi-static compliance measurements of WT and Vim −/− lungs. ( f ) Elastic modulus frequency plot obtained from live, unfixed lung tissue of saline and bleomycin-treated WT and Vim −/− animals. Microindentation data were fit using the Hertz model to acquire the elastic modulus of regions of lung tissue. Images in a – b represent data obtained from at least three animals per group; data shown in d – e are mean±s.d. of at least five animals. ** P <0.001, *** P <0.0001 relative to WT versus Vim −/− , by one-way analysis of variance with a correction provided by the Bonferroni multiple comparisons test. Full size image In patients with pulmonary fibrosis, pulmonary function tests typically reveal a parenchymal-restrictive ventilatory defect due to decreased lung compliance [36] . Lung compliance is influenced by the underlying connective tissue, which is rich in extracellular matrix components such as collagen [37] . Because Vim −/− mice exhibited less collagen deposition following treatment with either bleomycin or asbestos, we reasoned that lungs of these mice would maintain normal compliance. To test this hypothesis, we measured the lung mechanics of WT and Vim −/− mice using a SCIREQ ventilator 21 days following the bleomycin administration. In comparison with saline treatments, lungs of WT mice exhibited a 2.5-fold decrease in quasi-static compliance following the bleomycin administration, whereas the compliance of lungs from Vim −/− mice decreased only 1.3-fold ( Fig. 4e ). Bleomycin administration creates heterogeneous regions of lung fibrosis in mice ( Fig. 4a ), which is a pathologic feature of the human disease as well [38] . To assess focal changes in lung tissue stiffness, we performed regional nano-indentations on lung sections (200–400 μm thick) using atomic force microscopy (AFM). The micro-indentations provide a measure of the stiffness or elastic modulus ( E ) of lung tissue, which is inversely related to lung compliance. Elasticity maps from AFM micro-indentation from bleomycin-treated WT lungs clearly displayed the wide ranges of tissue stiffness ( Fig. 4c ), which corresponded to the heterogeneity of collagen deposition ( Fig. 4a ). The median elastic modulus of lung parenchymal tissue from WT mice increased 2.4-fold in response to bleomycin compared with control lung tissue (27 to 7.5 kPa, respectively), whereas the elastic modulus of lung tissue from bleomycin-treated Vim −/− mice was significantly decreased ( P <0.0001) compared with WT bleomycin-treated lung tissue ( Fig. 4f ). The wide range of E -values is reflected in the frequency of occurrence and in the median and interquartile ranges for each condition ( Supplementary Fig. 4b ). In addition, there was a strong correlation (Pearson r =−0.99) between the mean compliance values for each condition and the mean E -values for each condition (for example, WT-bleomycin-AFM versus WT-bleomycin-SCIREQ). Thus, the mechanical properties of the lung were preserved in Vim −/− mice following the bleomycin treatment, which is evident at both the global tissue scale and in focal regions of lung. Injury and fibrosis reduced in Vim−/− bone marrow chimeras Because multiple cell types contribute to the inflammatory and fibrotic responses, we next addressed the respective roles of bone marrow-derived cells in bleomycin-induced lung injury and fibrosis by generating bone marrow chimeras ( Fig. 5a ). Reconstitution of bone marrow from WT donor mice into irradiated recipient mice (WT) resulted in protein accumulation in BALF in response to bleomycin, whereas in recipient mice reconstituted with bone marrow from Vim −/− donor mice ( Vim −/− ), the BALF protein was unchanged from saline controls ( Fig. 5b ). Secretion of IL-1β ( Fig. 5c ), IL-6 ( Fig. 5d ) and TGF-β ( Fig. 5e ) in the BALF of WT mice significantly increased in response to bleomycin; the response in Vim −/− mice was significantly attenuated. Finally, WT mice displayed a significant degree of collagen deposition and fibrosis, as shown by Masson trichrome ( Fig. 5g ) and Picrosirius red stain ( Supplementary Fig. 5c ) and Sircol assay ( Fig. 5f ), whereas this response was severely attenuated in Vim −/− mice ( Fig. 5f,g and Supplementary Fig. 5c ). All together, these results suggest that vimentin-expressing bone marrow-derived cells are important for bleomycin-induced activation of the NLRP3 inflammasome and pulmonary fibrosis. 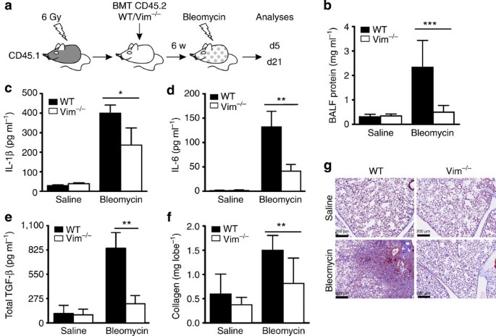Figure 5: Lung injury and fibrosis are attenuated inVim−/−bone marrow chimeric mice. (a) Treatment protocol: CD45.1+WT mice were lethally irradiated (6 Gy) and two sets of mice were transplanted either with 1 × 106CD45.2+WT orVim−/−BM cells to generate chimeric mice. After 6.5 weeks (w), when >90% of AM were of donor (WT andVim−/−) phenotype, chimeric mice were treated with saline or bleomycin and subjected to analyses. Bleomycin-induced lung injury was assessed by protein levels (b), and ELISA for IL-1β (c), IL-6 (d) and TGF-β (e) in BALF, 5 days (d5) after instillation. Bleomycin-induced fibrosis was assessed 21 days (d21) after instillation by measuring collagen content in lungs by Sircol assay (f) and by histological examination of lung tissue with H&E staining (g). Original magnification × 40; scale bar, 200 μm. Data inbare means±s.e.,c–fare means±s.d. from two independent experiments, each with at least three animals per experiment. *P<0.05, **P<0.001, ***P<0.0001, by one-way analysis of variance with a correction provided by the Bonferroni multiple comparisons test. Figure 5: Lung injury and fibrosis are attenuated in Vim −/− bone marrow chimeric mice. ( a ) Treatment protocol: CD45.1 + WT mice were lethally irradiated (6 Gy) and two sets of mice were transplanted either with 1 × 10 6 CD45.2 + WT or Vim −/− BM cells to generate chimeric mice. After 6.5 weeks (w), when >90% of AM were of donor (WT and Vim −/− ) phenotype, chimeric mice were treated with saline or bleomycin and subjected to analyses. Bleomycin-induced lung injury was assessed by protein levels ( b ), and ELISA for IL-1β ( c ), IL-6 ( d ) and TGF-β ( e ) in BALF, 5 days (d5) after instillation. Bleomycin-induced fibrosis was assessed 21 days (d21) after instillation by measuring collagen content in lungs by Sircol assay ( f ) and by histological examination of lung tissue with H&E staining ( g ). Original magnification × 40; scale bar, 200 μm. Data in b are means±s.e., c – f are means±s.d. from two independent experiments, each with at least three animals per experiment. * P <0.05, ** P <0.001, *** P <0.0001, by one-way analysis of variance with a correction provided by the Bonferroni multiple comparisons test. Full size image Loss of vimentin prevents NLRP3 activation As stated above, NLRP3 inflammasome activation requires two distinct stimuli. An inflammatory stimulus, such as LPS, primes cells to transcribe and synthesize pro-IL-1β (signal 1) and then another stimulus such as extracellular adenosine triphosphate (ATP), monosodium urate (MSU) or asbestos (signal 2) is necessary for inflammasome complex formation, caspase-1 activation and IL-1β maturation [19] , [22] , [39] . To further investigate the possibility that NLRP3 inflammasome activation requires vimentin, we isolated primary alveolar macrophages from WT and Vim −/− mice. Macrophages were primed with LPS and stimulated with ATP as previously described [39] . Levels of mature caspase-1 and IL-1β were significantly increased in the supernatants collected from WT macrophages following LSP and ATP treatment compared with saline treatment, but in the supernatant collected from Vim −/− macrophages there was only a slight increase ( Fig. 6a,b ). There was no difference in pro-IL-1β levels in total cell lysates between activated WT and Vim −/− alveolar macrophages ( Fig. 6c ; full blots are presented in Supplementary Fig. 7 ). As an independent approach, we expressed a small hairpin RNA (shRNA) targeted to vimentin (Vim KD ) or a scrambled shRNA (Ctrl) in J774a.1 macrophages and treated the cells with ATP. Caspase-1 is required to cleave pro-IL-1β into its biologically active form and like other caspases is proteolytically activated from a pro-enzyme to produce a tetramer of its two active subunits, p20 and p10 (ref. 28 ). The levels of mature caspase-1 p20, but not pro-caspase-1, were considerably reduced in Vim KD cells ( Fig. 6d,e ; full blots are presented in Supplementary Fig. 7 ) compared with Ctrl cells treated with ATP, further supporting the hypothesis that vimentin deficiency prevents NLRP3 inflammasome activation. 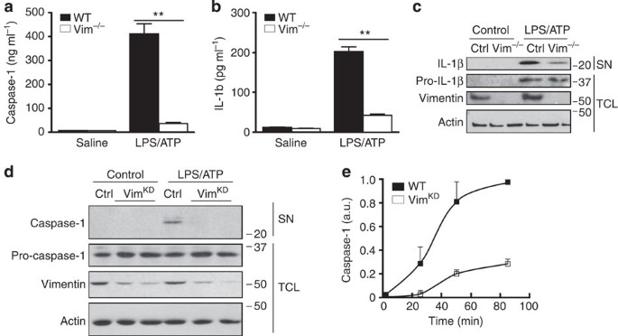Figure 6: Activation of the inflammasome in murine cells is dependent on vimentin. Primary WT andVim−/−alveolar macrophages were primed with LPS (100 ng ml−1) and treated with ATP (1 mM) or saline for 1 h. Caspase-1 (a) and IL-1β (b) levels in supernatants were assessed by ELISA and by western blot (c). J744.1 cells expressing either control shRNA (Ctrl) or shRNA against vimentin (KD, two distinct clones) were primed with LPS (100 ng ml−1) and treated with ATP (1 mM) or saline for 25 min. Vimentin, actin and caspase-1 protein levels were assessed by western blot analysis (d). Mature caspase-1 levels were assessed in WT and KD cells activated with ATP for 25, 50 or 85 min (e). Data shown are means±s.d. of three replicates. **P<0.001, by Student’st-test. SN, supernatant; TCL, total cell lysate. Figure 6: Activation of the inflammasome in murine cells is dependent on vimentin. Primary WT and Vim −/− alveolar macrophages were primed with LPS (100 ng ml −1 ) and treated with ATP (1 mM) or saline for 1 h. Caspase-1 ( a ) and IL-1β ( b ) levels in supernatants were assessed by ELISA and by western blot ( c ). J744.1 cells expressing either control shRNA (Ctrl) or shRNA against vimentin (KD, two distinct clones) were primed with LPS (100 ng ml −1 ) and treated with ATP (1 mM) or saline for 25 min. Vimentin, actin and caspase-1 protein levels were assessed by western blot analysis ( d ). Mature caspase-1 levels were assessed in WT and KD cells activated with ATP for 25, 50 or 85 min ( e ). Data shown are means±s.d. of three replicates. ** P <0.001, by Student’s t -test. SN, supernatant; TCL, total cell lysate. Full size image Uric acid released from cells exposed to bleomycin triggers NLRP3 inflammasome assembly leading to IL-1β maturation and inflammation in the lungs [19] , [40] . In an in vitro model, we examined whether silencing vimentin would impair NLRP3 inflammasome activation in response to MSU. A human macrophage-like cell line was treated with silencing RNA (siRNA) targeted to vimentin (Vim KD ) or a scrambled siRNA (CT; Fig. 7a ; full blots are presented in Supplementary Fig. 8 ) and subsequently activated with MSU. No differences were observed in the levels of pro-IL-1β between CT and Vim KD cells ( Fig. 7a ), suggesting that vimentin deficiency does not impair signal 1. NLRP3 inflammasome activation was repressed in Vim KD cells as assessed by IL-1β and caspase-1 levels in cell supernatants ( Fig. 7b,c ). Similar results were obtained when CT and Vim KD cells were activated with asbestos ( Fig. 7b,c ). In addition, bone marrow-derived macrophages (BMDMs) were isolated from WT and Vim −/− mice, primed with LPS and activated with MSU. Caspase-1 activation was assessed using a specific fluorescent probe, FAM-YVAD-FMK [41] . WT BMDMs showed robust caspase-1 activation following treatment with MSU, with caspase-1 forming aggregates throughout the cytoplasm. However, caspase-1 activation was severely reduced in BMDMs isolated from Vim −/− mice ( Fig. 7d ). No caspase-1 activation was observed in untreated BMDMs isolated from either WT or Vim −/− mice. 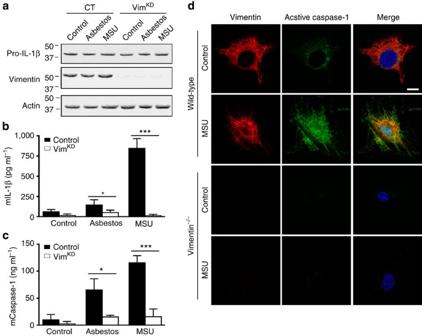Figure 7: Vimentin is required for inflammasome activationin vitro. Human THP-1 macrophages were differentiated and primed with PMA (0.5 μM) and treated with either scramble (CT) or vimentin (KD) siRNA and subsequently treated with saline, MSU (150 μg ml−1) or asbestos (40 μg cm−2) for 6 h. IL-1β, vimentin and actin levels in cell lysates were assessed by western blot (a), whereas levels of IL-1β (b) and caspase-1 (c) in supernatants were assessed by ELISA. (d) Confocal microscopy of BMDMs isolated from WT andVim−/−mice, primed with LPS as above, and activated with MSU (150 μg ml−1) for 3 h or left untreated. Cells were then labelled for active caspase-1 (green) according to manufacturer’s instructions, DNA (blue) and vimentin (red). Scale bar, 10 μm. Data shown are means±s.d., *P<0.05, ***P<0.0001, by one-way analysis of variance with a correction provided by the Bonferroni multiple comparisons test. Figure 7: Vimentin is required for inflammasome activation in vitro . Human THP-1 macrophages were differentiated and primed with PMA (0.5 μM) and treated with either scramble (CT) or vimentin (KD) siRNA and subsequently treated with saline, MSU (150 μg ml −1 ) or asbestos (40 μg cm −2 ) for 6 h. IL-1β, vimentin and actin levels in cell lysates were assessed by western blot ( a ), whereas levels of IL-1β ( b ) and caspase-1 ( c ) in supernatants were assessed by ELISA. ( d ) Confocal microscopy of BMDMs isolated from WT and Vim −/− mice, primed with LPS as above, and activated with MSU (150 μg ml −1 ) for 3 h or left untreated. Cells were then labelled for active caspase-1 (green) according to manufacturer’s instructions, DNA (blue) and vimentin (red). Scale bar, 10 μm. Data shown are means±s.d., * P <0.05, *** P <0.0001, by one-way analysis of variance with a correction provided by the Bonferroni multiple comparisons test. Full size image Vimentin interacts with inflammasome components Inflammasome activation involves the physical interaction of NLRP3, ASC (apoptosis-associated speck-like protein containing a CARD) and caspase-1 (ref. 28 ), but the mechanism by which the inflammasome assembles is not clear. If the vimentin network serves as a protein scaffold upon which the NLRP3 inflammasome components are assembled, then vimentin should interact with inflammasome proteins. Immunoprecipitation of caspase-1 and NLRP3 from human macrophage lysates resulted in a robust co-precipitation of vimentin, which was enhanced following activation of cells with ATP ( Fig. 8a ; full blots are presented in Supplementary Fig. 9 ). These interactions were specific for vimentin, as no actin was detectable in immunoprecipitates. 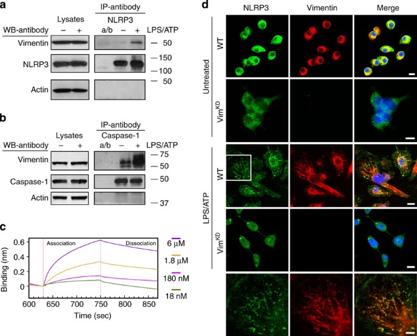Figure 8: Vimentin interacts with components of the NLRP3 inflammasome. Differentiated THP-1 cells primed with LPS (100 ng ml−1) and activated with ATP (2.5 mM) (a) or MSU (150 μg ml−1) (b) were immunoprecipitated. The presence of vimentin, actin and inflammasome proteins in immunoprecipitates was assessed by western blotting. In activated macrophages, vimentin co-immunoprecipitates with both NLRP3 and caspase-1, whereas actin does not. (c) The association between NLRP3 and vimentin was determined using a bio-layer interferometer (BLI). Various concentrations of vimentin were tested and representative association and dissociation curves are shown: 6 μM, purple; 1.8 μM, orange; 180 nM, pink; and 18 nM, green. (d) Vimentin (red) co-localizes with NLRP3 (green) in activated J774.1 macrophages treated with control shRNA, as assessed by confocal microscopy. Primed macrophages were either activated with ATP or left untreated before fixing and staining with anti-vimentin and anti-NLRP3 antibodies. Confocal images are representative of at least three independent experiments. Scale bar, 10 μm. Figure 8: Vimentin interacts with components of the NLRP3 inflammasome. Differentiated THP-1 cells primed with LPS (100 ng ml −1 ) and activated with ATP (2.5 mM) ( a ) or MSU (150 μg ml −1 ) ( b ) were immunoprecipitated. The presence of vimentin, actin and inflammasome proteins in immunoprecipitates was assessed by western blotting. In activated macrophages, vimentin co-immunoprecipitates with both NLRP3 and caspase-1, whereas actin does not. ( c ) The association between NLRP3 and vimentin was determined using a bio-layer interferometer (BLI). Various concentrations of vimentin were tested and representative association and dissociation curves are shown: 6 μM, purple; 1.8 μM, orange; 180 nM, pink; and 18 nM, green. ( d ) Vimentin (red) co-localizes with NLRP3 (green) in activated J774.1 macrophages treated with control shRNA, as assessed by confocal microscopy. Primed macrophages were either activated with ATP or left untreated before fixing and staining with anti-vimentin and anti-NLRP3 antibodies. Confocal images are representative of at least three independent experiments. Scale bar, 10 μm. Full size image We also used solution-binding assays to demonstrate a direct protein–protein interaction between vimentin and NLRP3. Bacterially expressed and purified S-tag His-vimentin was incubated with extracts prepared from either control or MSU-treated human macrophage cells. The S-tag vimentin was precipitated using S-protein agarose. The precipitated proteins were separated by sodium dodecyl sulfate polyacrylamide gel electrophoresis (SDS–PAGE), transferred to nitrocellulose and then immunoprobed with antibodies directed against NLRP3. We observed a 3.0±0.8-fold increase in binding between vimentin and NLRP3 in extracts prepared from MSU-treated cells, as compared with untreated control cells ( Supplementary Fig. 6 ). A complementary method, bio-layer interferometry (BLI), was also used to investigate the interaction between NLRP3 and vimentin. BLI is an optical technique that analyses the interference pattern of white light reflected from two surfaces: a layer of immobilized protein on the biosensor tip and an internal reference layer [42] . Any change in the number of molecules bound to the biosensor tip causes a shift in the interference pattern that can be measured in real time, providing detailed information on the kinetics of association and dissociation between the two molecules (k a , k d and K D ). Commercially available NLRP3 was bound to the biosensor tip, then various concentrations (55 μM, 18 μM, 6 μM, 1.8 μM, 180 nM, 18 nM and 1.8 nM) of full-length vimentin were added to determine the association kinetics with NLRP3. In agreement with other methods ( Fig. 8a,b,d and Supplementary Fig. 6 ), the assay demonstrated that NLRP3 binds to vimentin with a measureable affinity; a global dissociation constant (K D ) of 640 nM was determined using BLItz Pro. Consistent with the co-immunoprecipitation and solution-binding results, we observed co-localization of NLRP3 and vimentin in stimulated alveolar macrophages by confocal immunofluorescence microscopy ( Fig. 8d ). Following activation, the WT cells, but not the Vim KD cells, were spread and displayed lamellipodia. Furthermore, the vimentin network spanned the cytoplasm in the WT activated cells, whereas in unstimulated cells, the network appeared to be collapsed around the nucleus and lamellipodia were not observed ( Fig. 8d ). Vimentin filaments (red) strongly co-localized with NLRP3 (green) in both perinuclear and distal regions of the cells. Co-localization studies were performed using Fiji 1.48r (64-bit, win) and the Coloc 2 test [43] . Co-localization analyses were calculated on ROIs drawn around the lamellipodia, determined by the vimentin image. The thresholded Manders co-localization scores were 0.89±0.15 for vimentin and 0.86±0.18 for NLRP3. NLRP3 and ASC also co-localized in stimulated macrophages ( Supplementary Fig. 5 ); the score for NLRP3 co-localization with ASC in untreated cells was 0.20±0.11, indicating weak co-localization. In contrast, the score for NLRP3 co-localization with ASC in cells treated with ATP was 0.85±0.21, indicating strong co-localization. However, knockdown of vimentin resulted in a lack of co-localization between NLRP3 and ASC, even in activated macrophages ( Supplementary Fig. 5 ). Taken together, these results demonstrate that vimentin associates with components of the inflammasome and is required for inflammasome activation. Inflammation, the process aimed at restoring homeostasis after an insult, can be more damaging than the insult itself if uncontrolled, excessive or prolonged. Growing evidence indicates that IL-1β is a critical mediator of acute inflammation, remodelling and fibrosis in the lung. Using three well-characterized murine models of ALI and pulmonary fibrosis, which were previously shown to be dependent on the NLRP3 inflammasome [19] , [22] , [23] , [35] , we show that NLRP3 inflammasome activation, which leads to IL-1β maturation, is dependent on the type III IF protein vimentin. Our data obtained in vimentin knockout mice and vimentin-null cells suggest that vimentin is required for NLRP3 inflammasome activation. Dysregulated inflammation, excessive leukocyte accumulation and increased permeability of endothelial and alveolar epithelial barriers are the central pathophysiologic events in ALI and its most severe form, the acute respiratory distress syndrome (ARDS) [44] . All these end points were observed in WT mice challenged with LPS, bleomycin and asbestos. In contrast, Vim −/− mice exposed to the same treatments experienced mild increases in protein levels in BALF and limited alterations in lung histopathology, suggesting that they were protected from LPS-, bleomycin- and asbestos-induced ALI. Inflammasome-regulated cytokines have a key role in the initiation and propagation of the aforementioned features of ALI [45] . In fact, alveolar macrophages from patients with ARDS produce excessive amounts of IL-1β [46] , and IL-18 was elevated in the plasma of patients with ARDS, which correlated with increased morbidity and mortality [45] . Since vimentin-deficient mice were protected from ALI, we speculated that failure to produce inflammasome-mediated cytokines (for example, IL-1β) caused this protection. In fact, vimentin-deficient mice failed to increase mature IL-1β levels following exposure to LPS, asbestos or bleomycin. Moreover, we demonstrated that caspase-1 activation and mature IL-1β production in vitro requires vimentin, as no increase was observed in activated macrophages either isolated from Vim −/− mice or in which vimentin was silenced using RNA interference. Resolution of ALI/ARDS depends on a precise balance of inflammatory and molecular signalling [44] ; an imbalance in that process caused by IL-1β overproduction might prevent cellular restoration and lead to pulmonary fibrosis. In fact, IL-1β produced by the inflammasome has been recently identified as an initiator of fibrosis in response to bleomycin [35] , and administration of IL-1β alone recapitulates much of the lung pathology caused by bleomycin [47] . Because vimentin-deficient mice did not produce the same amount of IL-1β as WT mice, we reasoned that Vim −/− mice would be protected from bleomycin- and asbestos-induced pulmonary fibrosis. Indeed, lung pathology was significantly reduced in vimentin-deficient mice, pointing to the essential role of vimentin in pulmonary fibrosis. We found substantially less collagen deposition in Vim −/− mice compared with WT mice. The excessive collagen deposition in lungs of WT mice led to loss of mechanical compliance, whereas the lungs of Vim −/− mice maintained compliance similar to that of saline-treated mice. These results are consistent with previous reports demonstrating decreases in the compliance of fibrotic lungs [33] . The elastic modulus measurements strongly suggest that increased tissue stiffness at the microscale corresponds to areas of increased collagen deposition. Importantly, macroscale measurements of lung compliance were highly correlated with the microscale elastic modulus measurements obtained by AFM. A number of studies have demonstrated that IL-1β can induce ALI and contribute to the progression of pulmonary fibrosis [19] , [23] , [35] , [48] . IL-1β-induced fibrosis is associated with an increase in TGF-1β, demonstrating that ALI initiated by pro-inflammatory cytokines can result in progressive fibrosis [35] , [48] . Vim −/− mice were treated with recombinant mouse IL-1β (rmIL-1β 0.05 mg kg −1 body weight, intranasal (i.n. )), but we were unable to detect latent TGF-β1 in BALF from Vim −/− mice after i.n. rmIL-1β at days 1, 7 and 14 (data not shown), whereas latent TGF-β1 was detected 5 days after bleomycin administration in WT mice ( Fig. 3 ). Gasse et al. [19] reported that collagen deposition was increased by rmIL-1β in wild-type mice; Vim −/− mice treated with rmIL-1β had no increase in collagen deposition. We reason that the incomplete suppression of mIL-1β in Vim −/− mice is a reflection of incomplete chimera, with only ~90% engraftment. Studies with IL-1R1 −/− , MyD88 −/− , ASC −/− , Caspase-1 −/− and NLRP3 −/− mice have suggested that uric acid (induced by bleomycin), asbestos and silica are detected by the NLRP3 inflammasome in macrophages, likely leading to IL-1R1/MyD88 signalling in pulmonary epithelial cells, then to inflammation, neutrophil and lymphocyte recruitment and fibroblast activation [35] . Lung fibroblast activation results in collagen deposition and pulmonary fibrosis. Importantly, it was reported that vimentin is required for the stabilization of collagen mRNAs [49] . We reason that the Vim −/− mice treated with either rmIL-1β or WT bone marrow failed to increase collagen deposition because vimentin knockout fibroblasts fail to produce type I collagen due to decreased stability of collagen α1(I) and α2(I) mRNAs [49] . Protection from injury, inflammation and fibrosis has been observed in mice lacking any components of the NLRP3 inflammasome, similar to our observations of Vim −/− mice following injury [19] , [22] , [23] , [35] , [50] . These phenotypes led us to investigate whether vimentin might serve as a scaffold for the inflammasome by binding to one or more proteins in the inflammasome complex. Several studies have suggested that IFs, including vimentin, act as scaffolds for signalling molecules [2] , [11] , [12] . In fact, vimentin interacts with and is involved in the translocation of pERK1/2 to the nucleus [51] , limits the ability of 14-3-3 to interact with Raf and CdK1, and regulates the release and translocation of ROKα following RhoA activation. These findings exemplify how vimentin IFs can act as scaffolds for signalling molecules. Recently, vimentin was reported to bind to NOD2 (nucleotide-binding oligomerization domain-containing protein 2), a member of the NLR family, via the leucin-rich-repeat (LRR) [52] . The LRR is a protein-binding domain shared by 19 other NLR family members, including NLRP3. Therefore, we sought to determine whether vimentin interacts with NLRP3. In our experiments, immunoprecipitation of both NLRP3 and caspase-1 in lysates from WT alveolar macrophages resulted in a robust co-precipitation of vimentin, which was enhanced following activation of the NLRP3 inflammasome. These data were confirmed by immunofluorescent confocal microscopy of human and murine macrophages. The co-localization score for vimentin with NLRP3 was 0.89±0.15, indicating strong co-localization [43] . Moreover, we were able to demonstrate a direct protein–protein interaction between vimentin and NLRP3 by BLI assays, further establishing a role for vimentin in assembly of the NLRP3 inflammasome. Intermediate filaments, including vimentin, have been shown to provide a scaffold whereby active subunits of caspase-9 can activate caspase-3, which, in turn, can activate more caspase-9 resulting in an amplification loop [53] , [54] . Caspase-3, caspase-6 and caspase-7 have also been shown to interact with vimentin [54] ; to our knowledge, we are the first to report an interaction between caspase-1 and vimentin. We can only speculate about where and how vimentin associates with NLRP3 and caspase-1 during inflammasome assembly, since the crystal structures of the vimentin dimer and all components of the inflammasome except for PYD are unknown [13] , [14] , [15] . NLRP3 proteins have been shown to form inactive preassembled complexes in unstimulated cells [13] , [14] , [15] . Under stimulation, these proteins undergo conformational changes whereby the inflammasome is activated. The vimentin IF network could potentially associate with the NLRP3 inflammasome through one or more domains of NLRP3 and mediate the conformation change or stabilization of NLRP3 that leads to activation. We reason that vimentin may interact with NLRP3 in two distinct regions: the NACHT domain and the LRR; vimentin has been previously shown to interact with NOD2 in the LRR domain [52] . Because ASC is localized to the nucleus in unactivated cells, no interaction with vimentin is anticipated in nonactivated cells. Furthermore, on the basis of the structure of ASC, a PYD and CARD domain with a short linker, we do not anticipate a direct interaction with vimentin as vimentin lacks either of the ASC domains, therefore, any ASC signal following cell activation is anticipated to be due to vimentin interaction with other proteins in the inflammasome protein complex. An unresolved issue is how vimentin mediates inflammasome activation. Mitochondrial-derived reactive oxygen species (ROS) have been linked to inflammasome activation [55] . Vimentin IF are known to modulate mitochondrial motility [56] , and lack of vimentin results in increased ROS production [57] . This suggests that vimentin-deficient cells should have more robust inflammasome signalling, the exact opposite of what we have demonstrated. In a very provocative paper, however, Bauernfeind et al. [24] demonstrated that mitochondrial-derived ROS is required for priming, not activation, of the inflammasome, as ROS inhibitors blocked the priming step required for NLRP3 expression, but activation was not affected. This correlates with our findings that signal 1 is unaffected by the lack of vimentin. Further studies on the relationship between vimentin, mitochondria and ROS will likely provide insights into the regulation behind both signals 1 and 2 during inflammation, but currently they are beyond the scope of this paper. In summary, this study demonstrates a novel function for the type III IF, vimentin, in innate immunity and inflammation leading to ALI and pulmonary fibrosis. In our experiments, vimentin deficiency resulted in a blunted inflammatory response in the early stages of injury, which was consistent among the different animal models of lung injury used: LPS, bleomycin and asbestos. We further demonstrate that vimentin is required for IL-1β maturation through its interaction with the NLRP3 inflammasome. Vimentin may act as a scaffold for assembly of the inflammasome protein complex and thus regulate its function. Overall, this study provides new insights into lung inflammation and fibrosis, and importantly, suggests that vimentin may be a key regulator of the NLRP3 inflammasome. Mice and induction of acute lung injury Age- and sex-matched 8- to 10-week-old mice were used in all the experiments. The 129/Sv6 vimentin-deficient ( Vim −/− ) mice were a gift from Albee Messing (Madison, WI). Bleomycin (0.07 units in 50 μl of PBS; Hospira) and asbestos (200 μg in PBS; US EPA) were administered intratracheally via two 25-μl aliquots. LPS (80 mg kg −1 , lethal dose; 24 mg kg −1 , sublethal dose; Sigma-Aldrich) was administered via intraperitoneal injection. WT and Vim −/− mice were treated with a single intratracheal injection of 50 μl of phosphate-buffered saline (PBS) or bleomycin (0.07 units in 50 μl of PBS; Hospira). All mice were bred in our animal facility and the experiments were approved by the Northwestern University Animal Care and Use Committee. Histology A 20-gauge angiocath was sutured into the trachea, heart and lungs were removed en bloc and inflated with 0.8 ml of 4% paraformaldehyde. The heart and lungs were fixed and embedded in paraffin; 5-μm sections were stained with H&E, Picrosirius red or Masson trichrome [58] by the Mouse Histology Phenotyping Laboratory (Northwestern University, Chicago, IL). Sections were visualized using the TissueGnostics Tissue/Cell High Throughput Imaging Analysis System (Vienna, Austria) and captured using TissueFAXS software (TissueGnostics, Los Angeles, CA) at the Northwestern University Cell Imaging Facility. Specific regions of interest were visualized using a Zeiss Axioskop microscope and captured using the Cri NUANCE spectral camera software suite. Wet-to-dry weight ratios Mice were anaesthetised and lungs were surgically removed en bloc . The left lung was ligated, excised and weighed in a tared container. The left lung was then dried at 70 °C in a Speed-Vac SC100 evaporator (Thermo Scientific, Waltham, MA) until a constant weight was obtained, and the wet-to-dry weight ratio was calculated. Bronchoalveolar lavage To perform bronchoalveolar lavage (BAL), a 20-gauge angiocath ligated into the trachea and 1 ml of sterile PBS was instilled, then removed through the angiocath; the process was repeated three times. The samples were pooled and a 200 μl aliquot of the BAL fluid was placed in a cytospin and centrifuged at 500 g for 10 min. The pellet was re-suspended in 1 ml of PBS, plated on glass slides, stained with crystal violet and subjected to a blinded manual cell count and differential. Cytokine and chemokine levels in the supernatant were measured using the BD Cytometric Bead Array (BD Biosciences). Samples were analysed in triplicate using the Mouse Inflammation Kit (BD Biosciences) according to the instructions provided. This kit detects interleukin (IL)-6, MCP-1 and tumour necrosis factor (TNF)-α. Total transforming growth factor (TGF)-β1 was measured using the TGF-β1 RII DuoSet enzyme-linked immunosorbent assay (ELISA, R&D Systems, Minneapolis, MN) according to the manufacturer’s instructions. Total interleukin (IL)-1β was measured using the IL-β1 Ready-Set-GO ELISA (Ebioscience, San Diego, CA) according to the manufacturer’s instructions. Caspase-1 activity was measured using the Caspase-1 Fluorometric Assay (R&D Systems), according to the manufacturer’s instructions. Sircol assay Total collagen content was determined by harvesting lungs from mice 21 d after treatment with bleomycin or PBS, or 12 weeks after treatment with asbestos or TiO 2 . Exsanguination was accomplished by a left nephrectomy, followed by perfusion of the right ventricle with 2 ml of cold PBS. Both lungs were removed and homogenized (1 min with a tissue homogenizer followed by 12 strokes in a Dounce homogenizer) in 1 ml of 0.5 N acetic acid supplemented with Roche EDTA protease inhibitor. Aliquots of lung homogenate were then assayed for total lung collagen levels and compared with a standard curve prepared from rat tail collagen by using the Sircol collagen dye binding assay (BioColor Ltd, Newtownabbey, UK), according to the manufacturer’s directions. Compliance measurements WT and Vim −/− mice were anaesthetised with ketamine and xylazine (45 mg per 100 g of body weight) and a tracheotomy was performed. Pancuronium was administered intraperitoneally (0.08 μg kg −1 of body weight). The mouse was mechanically ventilated on a computer-controlled piston ventilator (FlexiVent; SCIREQ, Montréal, Québec, Canada) with a tidal volume of 10 ml kg −1 at a frequency of 150 breaths per minute against 2–3 cm H 2 O positive end-expiratory pressure. Following two total lung capacity manoeuvres to standardize volume history, pressure and flow data (reflective of airway and tissue dynamics) were collected during a series of standardized volume perturbation manoeuvres. These data were used to calculate both total lung resistance ( R ) and elastance ( E ) using the single-compartment model and used to derive further parameters of respiratory function. The FlexiVent calibration procedure removes cannula impedance from the reported data. Residual impedence ( I ) is therefore negligible and is not reported herein. Atomic force microscopy measurements Lungs were used at 17–21 days following bleomycin challenge. Following instillation of 2.5% low-gel point agar (50 ml kg −1 ), lungs were sectioned using a vibratome (Leica VT1000 S) into 200-μm or 400-μm thick slices. These slices were used within 24 h of harvest; micro-indentations were performed using a Bruker BioScope Catalyst located at the Northwestern University NUANCE facility. Modified probes with 5- μm spheres (Novascan, Ames, IA) were used to indent 80 μm × 80 μm areas on the lung slices. Force and indentation depth were converted to elastic modulus using the Hertz spherical indentation model [21] , [59] and a custom MATLAB program (generated by Dr Esra Roan, University of Memphis). A Poisson ratio of μ =0.4 was assumed for the tissue [60] , [61] , [62] . Cell culture To isolate bone marrow-derived macrophages (BMDM), bone marrow was extracted from mice femurs and tibia then purified through a Ficoll-Paque gradient. Upon purification, cells were differentiated on charge-free plates in DMEM containing 20% endotoxin-reduced fetal bovine serum and 30% L929 cell supernatant for 5 days [63] . Peritoneal macrophages were obtained from untreated mice. Briefly, the abdomen of anaesthetised mice was exposed and 5 ml of sterile PBS was instilled intraperitoneally using a 20-gauge syringe. Following agitation, the fluid was removed and centrifuged. The cells were plated in Dulbecco modified Eagle medium containing 10% fetal bovine serum and used for western blotting. Alveolar macrophages were obtained from BALF of untreated mice. Briefly, 1 ml of sterile PBS was instilled through a 20-gauge angiocath ligated into the trachea and the fluid then removed; this process was repeated three times. The fluid was centrifuged and cells were used for ELISA. The second-generation lentiviral pGIPZ expression vectors encoding shRNAs against mouse vimentin (clones V2LMM_14765, V2LHS_171946 and V2LHS_171949) and scrambled shRNA control (catalogue no. RHS4346) originated from the Thermo Fisher Scientific shRNA library (Waltham, MA) and were provided by RNAi/Throughput Robotics Core of Northwestern University (Evanston, IL). Lentiviral stocks (with titres of 10 7 –10 8 TU ml −1 ) encoding shRNAs against mouse vimentin were produced by the DNA/RNA Delivery Core (Skin Disease Research Center, Northwestern University, Chicago, IL). Western blotting Primary murine macrophages were cultured overnight in 1% serum and treated or not with LPS (100 ng ml −1 ) for 7 h. ATP (50 μM) was added to LPS-stimulated cells during the last 45 min. Cells were lysed in sample buffer and equal volumes loaded in 10% SDS–PAGE gels transferred to nitrocellulose membranes. The presence of indicated proteins in cell lysates and medium was assessed by western blotting using the following antibodies: mouse monoclonal anti-vimentin (clone V9; 1:500; Sigma-Aldrich no. V 6630, St Louis, MO), mouse monoclonal anti-NLRP3 (1:1,200, Adipogen International no. AG-20B-0014, San Diego, CA), chicken polyclonal anti-vimentin (1:500, Covance no. PCK-594P, Princeton, NJ), anti-pro-IL-1β, anti-IL-1β (clone p34; 1:1,000, Cell Signaling, Danvers, MA), anti-caspase-1 (1:1,000, Cell Signaling, no. 2225, Danvers, MA), and anti-actin (clone AC-15, 1:2,500, Sigma-Aldrich, St Louis, MO). Ponceau S staining was used to assess the release of total protein from activated macrophages. Membranes were blotted with antibodies as described in each figure. Untransfected J774.1 cells and two independent J774.1 clones expressing shRNAs against vimentin were primed with LPS (100 ng ml −1 ) for 5.5 h and then stimulated with ATP (1 mM) for 25, 50 or 85 min. Control cells (0) were incubated without ATP for 85 min. Immunocytochemistry The cells were grown on either collagen-coated coverslips or 35-mm glass-bottom dishes (MatTek Corp, Ashland, MA). Wild-type J774.1 cells and J774.1 cells expressing shRNA against vimentin were fixed in methanol (−20 °C) for 7 min and processed for indirect immunofluorescence as described previously [64] , [65] using the following antibodies: mouse monoclonal anti-NLRP3 (Adipogen International no. AG-20B-0014, San Diego, CA, 1:100 dilution), rabbit polyclonal anti-ASC (Adipogen International no. AG-25B-0006, San Diego, CA, 1:200 dilution), chicken polyclonal anti-vimentin (Covance no. PCK-594P, Princeton, NJ, 1:1,000 dilution), and appropriate secondary antibodies (Alexa Fluor 488 goat anti-mouse IgG, Alexa Fluor 568 goat anti-chicken IgG and Alexa Fluor 568 goat anti-rabbit IgG, Invitrogen no. A-11001, A-11041 and A-11011, respectively, Grand Island, NY, 1:200 dilution). Wild-type and Vim −/− BMDMs probed with FAM-YVAD-FMK (FAM-FLICA In Vitro Caspase Detection Kit, ImmunoChemistry, Bloomington, MN) were fixed in 2.7% paraformaldehyde for 15 min, permeabilized in 0.2% NP-40 for 3 min and processed for indirect immunofluorescence (rabbit polyclonal anti-vimentin, Cell Signaling no. 3932, Danvers, MA, 1:50 dilution; Alexa Fluor 568 goat anti-rabbit IgG, Invitrogen no. A-11011, Grand Island, NY, 1:200 dilution). Images of fixed, stained preparations were taken with either a Zeiss LSM 510 microscope or a Nikon A1R microscope. Some images were contrast enhanced using Zeiss LSM Image software. Protein precipitation THP-1 cells were differentiated with PMA (50 nM) for 48 h, followed by 72 h of incubation in complete medium. The cells were cultured overnight in 1% serum in DMEM with pen/strep and treated or not with LPS (100 ng ml −1 ) for 6 h. ATP (50 μM) was added to LPS-stimulated cells during the last 45 min. Cell lysates were cleared by centrifugation and immunoprecipitated overnight (IP) with antibodies directed against NLRP3 (mouse monoclonal anti-NLRP3, 1:100, Adipogen International no. AG-20B-0014, San Diego, CA) or caspase-1 (1:1,000, Cell Signaling, Danvers, MA). Immunoprecipitated caspase-1 in the right panel could not be detected due to masking by the signal from the heavy chain of the antibody. Protein A/G agarose was incubated with cell lysates in the absence of an antibody to control for non-specific binding. To enable caspase-1 detection in immunoprecipitates, caspase-1 antibodies were crosslinked to protein A/G agarose using Crosslink IP kit (Thermo). Protein A/G agarose beads were used for immunoprecipitation, in some cases the antibody used for IP was crosslinked to the beads (Thermo). Immunoprecipitated proteins were eluted with a low pH buffer and precipitated with ethanol. The buffer used was as follows: 20 mM HEPES (pH 7.5), 100 mM NaCl, 1 mM EGTA, 5 mM MgCl2, 0.5% sodium deoxycholate, 0.5% TX-100, 10 μg ml −1 TPCK, 2 μg ml −1 leupeptin, 0.1 mM PMSF, phosphatase inhibitor cocktail (1:200 dilution, Sigma), 0.1 mM sodium orthovanadate. In other experiments, Vim −/− BMDM cell extracts were prepared by lysis on ice using 25 mM Tris pH 7.4, 150 nM NaCl, 1 mM EDTA, 1% NP-40 and 5% glycerol and protease inhibitors (Roche). The extracts were clarified at 14,000 g for 15 min at 4 °C. To 2 mg of cell extract, 20 μg of bacterially expressed and purified S-tag, His-tag vimentin was added and incubated at 4 °C for 16 h to precipitate vimentin and bound proteins. Then washed S-protein agarose beads (EMD Millipore) were added to the mixture and rotated at 25 °C for 30 min. The beads were treated according to manufacturer’s instructions. Bound proteins were prepared for western blotting. Protein–protein interaction The interaction between NLRP3 and vimentin was analysed using a BLI, BLItz (ForteBio, Menlo Park, CA). Antibodies directed against NLRP3 (Adipogen) were diluted 1:4 then attached to a protein A biosensor. Next, commercially available, purified NLRP3 (Abnova) was attached to the biosensor for 3 min. Finally, each labelled biosensor was placed into a specific concentration of purified vimentin [66] and binding was measured for 120 s followed by dissociation in PBS for 120 s. At the start of each binding experiment, vimentin was diluted into PBS to assemble filaments [67] . After multiple experiments, the association and dissociation constants of all experiments were globally fitted to determine a value of K D for vimentin interacting with NLRP3 using the BLItz Pro software version 1.1.0.29. Mouse chimeras Recipient mice (B6.SJL-Ptprc[d]Pep3[a]/BoyJ [B6.SJL] [PepBoy]) underwent a single lethal total body irradiation. Fresh bone marrow cells (5 × 10 6 cells per mouse) from WT 129S/v6 or Vim −/− 129S/v6 donor mice were injected into the lateral tail vein of the irradiated recipient mice within 24 h following a single total body irradiation of 10.5 Gy. The reconstituted mice were used 39–45 days after bone marrow transplantation. The protocol resulted in ~90% of blood circulating leukocytes of donor origin as assessed by percentage of CD45.1+ and CD45.2+ cells in the peripheral blood using flow cytometry. Real-time reverse transcriptase polymerase chain reaction Total RNA extraction and quantitative PCR were performed as previously described (). Briefly, total RNA was isolated using the Aurum Total RNA mini kit (Qiagen). cDNA was synthesized using the qScript cDNA Supermix (Quanta Biosciences) and amplified using 40-cycle two-step PCR with sequence-specific primer pairs (IDT). SYBR Green fluorescence was quantified with a CFX96 Real-Time System Thermal Cycler (Bio-Rad) using ΔΔ C T analysis. Relative IL-1β mRNA expression was determined via normalizing to β-actin mRNA expression. Statistical analysis Data are expressed as means±s.d. or means±s.e.m. Differences between two groups were assessed by using a Student’s t -test. Differences between three or more groups were assessed using one-way analysis of variance with a Bonferroni multiple comparisons test. Values of P <0.05 were considered to be significant. The log rank test, which calculates the chi-square ( χ 2 ) for each event time for each group and sums the results, was used in the analysis of the Kaplan–Meier curve was used. All analyses were performed using GraphPad Prism software version 4.00 for Windows (GraphPad Software, San Diego, CA). How to cite this article: dos Santos, G. et al. Vimentin regulates activation of the NLRP3 inflammasome. Nat. Commun. 6:6574 doi: 10.1038/ncomms7574 (2015).